The CD4+T-cell help signal is transmitted from APC to CD8+T-cells via CD27–CD70 interactions CD8 + cytotoxic T lymphocytes are critical components of immunity against infectious pathogens, tumours, and in the case of pathogenic autoimmunity, normal self tissues. CD4 + T (T H ) cells provide 'help' to CD8 + cytotoxic T lymphocytes during priming by first activating antigen-presenting cells via CD40–CD40L interactions. Here we show that, after immunization with either a noninflammatory, nonreplicating antigen or an overtly inflammatory replicating antigen, CD8 + cytotoxic T lymphocytes prevented from receiving a signal through CD27 during priming subsequently exhibit a specific defect in their capacity for secondary expansion that can be rescued by the absence of TRAIL. Thus, the 'help message' is transmitted to CD8 + T cells via CD70–CD27 signals, enabling them to undergo secondary expansion and avoid TRAIL-mediated apoptosis on re-stimulation. These findings complete our understanding of the cellular interactions through which T H is provided to CD8 + cytotoxic T lymphocytes during priming. CD8 + cytotoxic T lymphocytes (CTL) are critical in the control of bacterial and viral pathogens, and can have a key role in the control of tumours as well as rejection of tissue grafts [1] . CD4 + 'helper' T cells (T H cells) have several important roles during the development and maintenance of CTL responses, including the enhancement of clonal expansion during priming, facilitating the entry of effectors into inflamed tissues, and promoting the long-term homeostatic survival of memory cells [1] , [2] , [3] , [4] . Before exerting these functions, however, T H cells must catalyse the functional activation of antigen-presenting cells (APC) to a state in which they can autonomously prime memory CTL capable of secondary expansion. Numerous studies have established a role for CD40-L-CD40 interactions in T H -mediated APC activation; yet, little information is known about the signals provided by activated APC that allow the help message to be transmitted to the CTL during priming [5] . To aid in defining these signals, we and others have established specific phenotypic and functional characteristics by which 'helped' memory CTL can be identified. These include the capacity for secondary expansion on antigenic stimulation and avoidance of the TRAIL-mediated activation-induced cell death (AICD) that occurs in 'helpless' CTL (those primed in the absence of T H cells) [6] , [7] , [8] , [9] . These distinct outcomes to secondary stimulation of daughter cells seem to be 'programmed' in their clonal precursors, that is, directed by a genetic program that is defined by the range of signals received during priming [10] . We therefore sought to investigate the costimulatory ligands induced in APC by CD40 engagement that can generate positive signals capable of conferring this functional capacity through receptors expressed on naïve CTL. The CD27–CD70 receptor/ligand pair is of interest in this regard, as members of the TNF-receptor superfamily (TNFSF) have been shown to control growth and survival of T cells [11] . CD27 is expressed on naïve CTL, as well as CD4 + T cells, natural killer (NK) cells and a subset of B cells, and expression of its one known ligand, CD70 can be induced on dendritic cells by the combined stimulation of inflammatory [12] and T H -mediated pathways (via CD40) [12] , [13] , [14] , [15] . Several lines of evidence suggest that CD70 induction is an important functional downstream consequence of T H -mediated dendritic cell (DC) activation, and that engagement of CD27 on CTL represents a crucial step in their acquisition of the memory state. First, upregulation of CD70 on DC—either by CD40-activation, inflammatory stimuli, or through transgenic expression, is directly associated with their ability to prime both effector and memory CTL, as well as reversing tolerance to self-antigen [12] , [14] , [16] , [17] . Conversely, blockade of CD70 blunts the induction of CTL when measured as either primary effectors or memory cells [14] , [18] , [19] . Lastly, the absence of CD27 on CD8 + T cells has been shown to profoundly diminish the generation and maintenance of both effector and memory CTL in some, but not all, models of viral infection, suggesting that either inflammation and/or antigen persistence may have a role in determining the requirement for this pathway [18] , [20] , [21] , [22] , [23] , [24] . Although these studies make clear that the CD27/CD70 pathway can have a crucial role in CTL priming, they reveal variability in its requirement depending on the nature of the immunogen and do not unambiguously specify a role for CD27 in communicating the help message to CTL. To overcome these issues, we have assessed the role of CD27–CD70 interactions in the primary and secondary CTL response to both replicating and nonreplicating immunogens using an in vivo system in which the expression of CD27 can be manipulated exclusively on the responding CTL. We find that CD27 transmits the signals that endow CTL with the capacity for secondary expansion and avoidance of TRAIL-mediated AICD on re-encounter with antigen. CD70 blockade leads to defective secondary CTL expansion We sought to determine the influence of CD27–CD70 signals provided during the priming on the subsequent generation of primary and secondary CTL responses against replicating and nonreplicating immunogens. This was initially accomplished by administration of a blocking antibody against CD70, during the first 3 days, after infection of intact and CD4-depleted mice with a recombinant vaccinia virus expressing the model antigen chicken ovalbumin (Vacc-OVA). We first confirmed that CD70 expression was slightly higher on CD11c + APC from intact mice than those depleted of T H cells ( Fig. 1a ). Antibody-mediated blockade of CD70 during priming produced a slight reduction in the magnitude of the antigen-specific primary CTL response measured at day 7, with comparable numbers of memory cells detected at day 45 in both intact (helped) and CD4-depleted (helpless) conditions ( Fig. 1b–e ). The magnitude of secondary expansion, following antigenic challenge with Listeria monocytogenes OVA (LM-OVA), whether measured at day 45 by their relative frequency or absolute number, was reduced in intact mice in which CD70 had been blocked during priming to a level that was comparable with that observed in de facto 'helpless' CTL primed in the absence of T H cells. The same result was observed following Vacc-OVA challenge of mice immunized with a noninflammatory, nonreplicating immunogen expressing the same antigen: Act-mOVA/K b−/− splenocytes that depend on cross-priming by host APC for their generation due to the lack of the appropriate MHC class I molecule required for direct presentation of the OVA 257−264 peptide to CTL ( Fig. 1f,g ). No effect on secondary expansion was seen when CD70 was blocked during the challenge phase of mice primed with Act-mOVA/K b−/− splenocytes ( Fig. 1h,i ). These findings show that blockade of CD70 during priming programs the resulting CTL to undergo a phenotypically 'helpless' response that is characterized by a defective secondary expansion, despite the availability of demonstrably effective CD4 + T cell help. 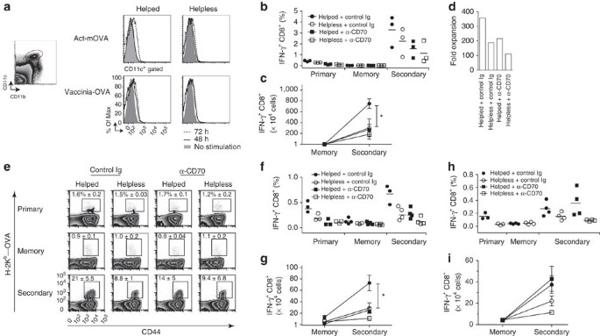Figure 1: CD70 blockade results in defective secondary T-cell expansion. (a) Groups of 3–4 WT mice were treated with the anti-CD4 antibody GK1.5 to deplete CD4+ cells 3 days (200 μg per mouse) and 1 day (100 μg per mouse) before immunization with either 5×106Act-mOVA/Kb−/−splenocytes or 106pfu Vacc-OVA. CD70 expression was then measured on CD11c+cells, by flow cytometry, 48 and 72 h later. (b–e). Groups of 3–4 intact (filled symbols) or CD4-depleted (open symbols) WT mice were treated with 250 μg per mouse of the CD70 blocking antibody FR70 (squares) or control antibody (circles) at day −1, 0 and 3 after infection with Vacc-OVA. Forty days later, mice were challenged with 0.6 LD50L.M.-OVA. OVA257−264/Kb-specific CTL were enumerated by MHC/peptide tetramer analysis and IFN-γ ICS at day 7 (primary), and day 45 in mice that either had (secondary) or had not (memory) received the LM-OVA challenge 5 days earlier. (b) Percentage of IFN-γ+CD8+ among total splenocytes and (c) their absolute number. Error bars represent s.d. within each group. (d) X-fold expansion from (c) of the OVA257−264/Kb-specific CTL enumerated by IFN-γ ICS in mice treated (or not) with CD70-blocking antibody (fold expansion is the ratio of the absolute number of OVA257−264/Kb-specific CTL at the memory phase to the one at the secondary response). (e) Dot plots of the % tetramer+CTL among the CD8+T cell population and the average value per group. (f,g) Mice were treated with FR70 or control antibody as above following priming with Act-mOVA/Kb−/−splenocytes and challenged at day 40 with 5×106pfu Vacc-OVA, and primary, memory and secondary OVA-specific CTL were measured by IFN-γ ICS, as described above. (f) Percentage of IFN-γ+CD8+among total splenocytes and (g) their absolute number. (h,i) Groups of 3–4 intact (filled symbols) or CD4-depleted (open symbols) mice were immunized with Act-mOVA/Kb−/−splenocytes and treated 29 days later with FR70 (squares) or isotype control antibody (circles) at day 0, 1 and 3 after infection with 5×106pfu Vacc-OVA. OVA-specific CTL were enumerated by IFN-γ ICS at day 7 (primary), and day 34 in mice that either had (secondary) or had not (memory) received Vacc-OVA challenge 5 days earlier. (h) Percentage of IFN-γ+CD8+ among total splenocytes and (i) their absolute number. Significant difference was calculated by an unpaired two-tailedt-test. *P-value<0.05. The figures show representative experiments that were repeated at least twice with similar results. Figure 1: CD70 blockade results in defective secondary T-cell expansion. ( a ) Groups of 3–4 WT mice were treated with the anti-CD4 antibody GK1.5 to deplete CD4+ cells 3 days (200 μg per mouse) and 1 day (100 μg per mouse) before immunization with either 5×10 6 Act-mOVA/K b−/− splenocytes or 10 6 pfu Vacc-OVA. CD70 expression was then measured on CD11c + cells, by flow cytometry, 48 and 72 h later. ( b–e ). Groups of 3–4 intact (filled symbols) or CD4-depleted (open symbols) WT mice were treated with 250 μg per mouse of the CD70 blocking antibody FR70 (squares) or control antibody (circles) at day −1, 0 and 3 after infection with Vacc-OVA. Forty days later, mice were challenged with 0.6 LD50L.M.-OVA. OVA 257−264 /K b -specific CTL were enumerated by MHC/peptide tetramer analysis and IFN-γ ICS at day 7 (primary), and day 45 in mice that either had (secondary) or had not (memory) received the LM-OVA challenge 5 days earlier. ( b ) Percentage of IFN-γ+CD8+ among total splenocytes and ( c ) their absolute number. Error bars represent s.d. within each group. ( d ) X-fold expansion from ( c ) of the OVA 257−264 /K b -specific CTL enumerated by IFN-γ ICS in mice treated (or not) with CD70-blocking antibody (fold expansion is the ratio of the absolute number of OVA 257−264 /K b -specific CTL at the memory phase to the one at the secondary response). ( e ) Dot plots of the % tetramer + CTL among the CD8 + T cell population and the average value per group. ( f , g ) Mice were treated with FR70 or control antibody as above following priming with Act-mOVA/K b−/− splenocytes and challenged at day 40 with 5×10 6 pfu Vacc-OVA, and primary, memory and secondary OVA-specific CTL were measured by IFN-γ ICS, as described above. ( f ) Percentage of IFN-γ + CD8 + among total splenocytes and ( g ) their absolute number. ( h , i ) Groups of 3–4 intact (filled symbols) or CD4-depleted (open symbols) mice were immunized with Act-mOVA/K b−/− splenocytes and treated 29 days later with FR70 (squares) or isotype control antibody (circles) at day 0, 1 and 3 after infection with 5×10 6 pfu Vacc-OVA. OVA-specific CTL were enumerated by IFN-γ ICS at day 7 (primary), and day 34 in mice that either had (secondary) or had not (memory) received Vacc-OVA challenge 5 days earlier. ( h ) Percentage of IFN-γ + CD8+ among total splenocytes and ( i ) their absolute number. Significant difference was calculated by an unpaired two-tailed t -test. * P -value<0.05. The figures show representative experiments that were repeated at least twice with similar results. Full size image CD27 is required to generate 'helped' CTL We next evaluated the effect of global CD27 deficiency on primary and secondary CTL expansion in response to replicating and nonreplicating immunogens. CD27 −/− mice displayed a reduced primary response, as measured by either OVA 257−264 /K b tetramer or ICS analysis, compared with wild-type controls following immunization with either Vacc-OVA or Act-mOVA/K b−/− splenocytes, although comparable numbers of memory cells were detectable at day 45 in both hosts ( Fig. 2a–c ). Following challenge with LM-OVA, however, the intact CD27 −/− mice showed a specific defect in secondary CTL expansion that was equivalent to that seen in wild-type mice lacking T H cells ( Fig. 2b ). The same pattern of defective and phenotypically 'helpless' secondary expansion was observed in CD27 −/− mice immunized with Act-mOVA/K b−/− splenocytes, although the decrease in primary response magnitude was not as pronounced with the nonreplicating immunogen that itself was substantially dependent on the presence of CD4 + T cells ( Fig. 2d,e ). Taken together, these data indicate that the dependence on T H cells and CD27 expression for optimal primary CTL responses can vary based on the nature of the immunogen, that is, an infectious replicating versus nonreplicating antigen, but that secondary expansion requires that both be present during priming. 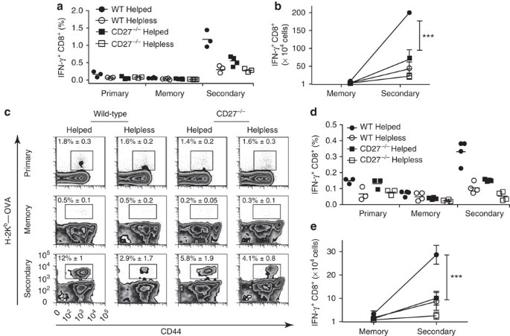Figure 2: Absence of CD27 results in defective secondary expansion. (a–c) Groups of 3–4 intact (filled symbols) or CD4-depleted (open symbols) C57BL/6 mice (circles) or CD27−/−mice (squares) were infected with 1×106pfu Vacc-OVA. Forty days later, some groups were challenged with 0.6 LD50L.M.-OVA. OVA257−264/Kb-specific CTL were enumerated by Kb/OVA257−264tetramer analysis and by IFN-γ ICS at day 7 (primary) and day 45 in mice that either had (secondary) or had not (memory) received the LM-OVA challenge 5 days earlier. (a) The percentage of IFN-γ+CD8+among total splenocytes and (b) their absolute number. Error bars represent s.d. within each group. (c) Dot plots of the % tetramer+ CTL among the CD8+T-cell population with the numbers in each panel depicting the average value per group. (d,e) Mice were primed with 5×106Act-mOVA/Kb−/−splenocytes and challenged at day 40 with 5×106pfu Vacc-OVA and primary, memory and secondary OVA257−264/Kb-specific CD8+ T cell was measured by IFN-γ ICS, as described above. (d) The % of IFN-γ+CD8+among total splenocytes and (e) their absolute number. Significant difference was calculated by an unpaired two-tailedt-test. *P-value<0.05; **P<0.005; ***P<0.0005. The data show representative experiments that were repeated at least twice with similar results. Figure 2: Absence of CD27 results in defective secondary expansion. ( a – c ) Groups of 3–4 intact (filled symbols) or CD4-depleted (open symbols) C57BL/6 mice (circles) or CD27 −/− mice (squares) were infected with 1×10 6 pfu Vacc-OVA. Forty days later, some groups were challenged with 0.6 LD50L.M.-OVA. OVA 257−264 /K b -specific CTL were enumerated by Kb/OVA 257−264 tetramer analysis and by IFN-γ ICS at day 7 (primary) and day 45 in mice that either had (secondary) or had not (memory) received the LM-OVA challenge 5 days earlier. ( a ) The percentage of IFN-γ + CD8 + among total splenocytes and ( b ) their absolute number. Error bars represent s.d. within each group. ( c ) Dot plots of the % tetramer+ CTL among the CD8+T-cell population with the numbers in each panel depicting the average value per group. ( d , e ) Mice were primed with 5×10 6 Act-mOVA/K b−/− splenocytes and challenged at day 40 with 5×10 6 pfu Vacc-OVA and primary, memory and secondary OVA 257−264 /K b -specific CD8+ T cell was measured by IFN-γ ICS, as described above. ( d ) The % of IFN-γ + CD8 + among total splenocytes and ( e ) their absolute number. Significant difference was calculated by an unpaired two-tailed t -test. * P -value<0.05; ** P <0.005; *** P <0.0005. The data show representative experiments that were repeated at least twice with similar results. Full size image CTL require CD27 expression for secondary expansion Given the number and variety of cells expressing CD27, it became important to determine whether its demonstrated requirement in secondary CTL expansion was cell-intrinsic. This involved first evaluating the need for CD27 expression on CD4 + T cells for their ability to transmit help using an in vivo system in which a defined population of Ag-specific helper cells enables the primary and secondary response of endogenous CTL. A discrete population of wild-type or CD27-deficient OVA 323−339 /I-A b -specific OT-II CD4 + T cells was first transferred to CD4 −/− mice. One day later, these mice were immunized with Act-mOVA/K b−/− splenocytes and the primary response of the endogenous CTL response was measured 7 days afterwards ( Fig. 3a,b ). As seen in Fig. 3 , the primary and memory CTL response is heavily dependent on the provision of CD4 + T cell help in this system. The same outcome was observed for secondary responses when the mice were challenged with Vacc-OVA 30 days later in that CD4 + T cells were clearly required to provide help during priming but importantly, they do not require expression of CD27 to do so ( Fig. 3c ). These data reveal that, in contrast to that reported for protein immunization, the absence of CD27 on the CD4 + T cells did not hamper their ability to provide help for CTL responding to a cellular vaccine [25] . 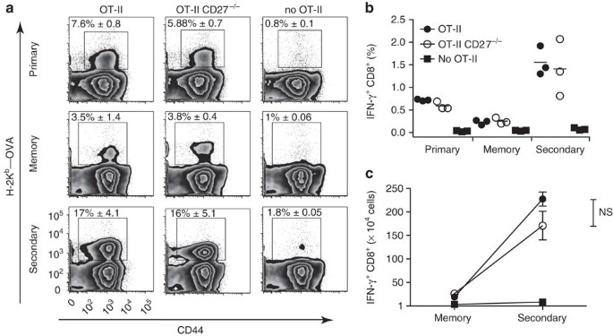Figure 3: CD4+T cells do not require CD27 expression to provide help. Groups of 4 CD4−/−mice received 5×104wild-type or CD27−/−OT-II cells. One day later, the mice were challenged with 5×106Act-mOVA/Kb−/−splenocytes. After 7 days, the primary endogenous OVA257−264/Kb-specific response was measured by MHC/peptide tetramer analysis and intracellular cytokine staining for IFN-γ. Some groups were re-challenged 30 days later with 5×106pfu Vacc-OVA and the secondary response measured 5 days later. (a) The percentage of IFNγ+OVA257−264/Kb-specific CD8+among total splenocytes spleen during primary (day 7), memory (day 30) and secondary response (day 30+5 days post challenge). (b) The absolute number of IFNγ+OVA257−264/Kb-specific CTL in the spleen, and (c) the OVA OVA257−264/Kb-specific/Kbtetramer response by the CTL at these same time points. Error bars represent the s.d. of three mice. Significant difference was calculated by an unpaired two-tailedt-test. *P-value<0.05; **P<0.005; ***P<0.0005. The figures show representative experiments that were repeated at least twice with similar results. Figure 3: CD4 + T cells do not require CD27 expression to provide help. Groups of 4 CD4 −/− mice received 5×10 4 wild-type or CD27 −/− OT-II cells. One day later, the mice were challenged with 5×10 6 Act-mOVA/K b−/− splenocytes. After 7 days, the primary endogenous OVA 257−264 /K b -specific response was measured by MHC/peptide tetramer analysis and intracellular cytokine staining for IFN-γ. Some groups were re-challenged 30 days later with 5×10 6 pfu Vacc-OVA and the secondary response measured 5 days later. ( a ) The percentage of IFNγ + OVA 257−264 /K b -specific CD8 + among total splenocytes spleen during primary (day 7), memory (day 30) and secondary response (day 30+5 days post challenge). ( b ) The absolute number of IFNγ + OVA 257−264 /K b -specific CTL in the spleen, and ( c ) the OVA OVA 257−264 /K b -specific/K b tetramer response by the CTL at these same time points. Error bars represent the s.d. of three mice. Significant difference was calculated by an unpaired two-tailed t -test. * P -value<0.05; ** P <0.005; *** P <0.0005. The figures show representative experiments that were repeated at least twice with similar results. Full size image We next investigated the role of CD27 on CTL using a similar adoptive transfer approach in which expression could be selectively manipulated on the relevant antigen-specific CTL population. Groups of intact or CD4-depleted C57BL/6 mice received 50 OT-I or OT-I CD27 −/− CTL, and were subsequently infected one day later with Vacc-OVA. Whether the two OT-I populations were transferred either singly or together, the primary and secondary responses (measured following challenge with LM-OVA) were decreased when CD27 was absent from these cells ( Fig. 4a–e ). Importantly, the relative frequency of memory cells before challenge was comparable between the two CTL populations, indicating that a specific defect in the capacity for secondary expansion results from the specific absence of CD27 on CD8 + T cells ( Fig. 4e ). This was confirmed in radiation bone-marrow chimeras constructed using equal numbers of congenic wild-type or CD27 −/− bone marrow ( Fig. 4f ), demonstrating that this effect is also true for endogenous polyclonal responders. The range of values obtained for the primary response to Vacc-OVA is similar to previous data published [26] . These findings confirm that the CTL themselves must express CD27 to receive the requisite signals needed for their subsequent optimal secondary expansion. 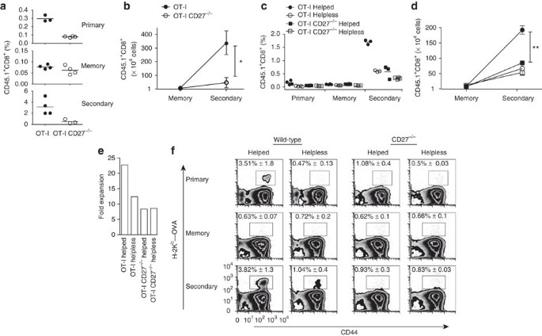Figure 4: CD27 expression on CTL is required for secondary expansion. (a,b) Groups of 4 C57BL/6 (CD45.2+) mice received 50 WT (filled circles) or CD27−/−(open circles) CD45.1+OT-I CTL. One day later, the mice were infected with 1×106pfu Vacc-OVA. 40 days later, some groups were challenged with 0.6 LD50L.M.-OVA. The response magnitude of each OT-I population measured by enumerating CD45.1+cells among total splenocytes at day 7 (primary), and day 45 in mice that either had (secondary) or had not (memory) received the LM-OVA challenge 5 days earlier. (a) The percentage of OT-I CD8+among total splenocytes with the average value depicted by the horizontal line, and (b) their absolute number. Error bars represent the standard deviation within each group. (c,e) Groups of 4 intact (filled symbols) or CD4-depleted (open symbols) C57BL/6 mice received 50 wild-type OT-I (circles, CD45.1+/2+) and 50 CD27−/−OT-I (squares, CD45.1+) CTL and then primed and challenged as above in (a). (c) The % of OT-I CD8+among total splenocytes with the average value depicted by the horizontal line and (d) their absolute number. (e) The fold expansion from (d) of the OT-I CD8+ T cells. Significant difference was calculated by an unpairedt-test. (f) Mixed bone-marrow chimeras were generated in lethally irradiated (1100R) C57BL/6J hosts reconstituted with a 50:50 mix of wild-type (CD45.1+) and CD27−/−(CD45.2+) T-cell-depleted bone-marrow cells. Eight weeks after reconstitution, the chimeras were primed with 5×106Act-mOVA/Kb−/−splenocytes and challenged at day 40 with 5×106pfu Vacc-OVA. The frequency of OVA257−264/Kb–specific CTL of each type at primary, memory and following secondary expansion in the presence (helped) versus absence (helpless) of CD4+T cells is shown. Standard error bars represent the s.d. of mice in each group. Significant difference was calculated by an unpaired two-tailedt-test. *P-value<0.05; **P<0.005; ***P<0.0005. Figure shows representative experiments that were repeated at least twice with similar results. Figure 4: CD27 expression on CTL is required for secondary expansion. ( a , b ) Groups of 4 C57BL/6 (CD45.2 + ) mice received 50 WT (filled circles) or CD27 −/− (open circles) CD45.1 + OT-I CTL. One day later, the mice were infected with 1×10 6 pfu Vacc-OVA. 40 days later, some groups were challenged with 0.6 LD50L.M.-OVA. The response magnitude of each OT-I population measured by enumerating CD45.1 + cells among total splenocytes at day 7 (primary), and day 45 in mice that either had (secondary) or had not (memory) received the LM-OVA challenge 5 days earlier. ( a ) The percentage of OT-I CD8 + among total splenocytes with the average value depicted by the horizontal line, and ( b ) their absolute number. Error bars represent the standard deviation within each group. ( c , e ) Groups of 4 intact (filled symbols) or CD4-depleted (open symbols) C57BL/6 mice received 50 wild-type OT-I (circles, CD45.1 + /2 + ) and 50 CD27 −/− OT-I (squares, CD45.1 + ) CTL and then primed and challenged as above in ( a ). ( c ) The % of OT-I CD8 + among total splenocytes with the average value depicted by the horizontal line and ( d ) their absolute number. ( e ) The fold expansion from ( d ) of the OT-I CD8+ T cells. Significant difference was calculated by an unpaired t -test. ( f ) Mixed bone-marrow chimeras were generated in lethally irradiated (1100R) C57BL/6J hosts reconstituted with a 50:50 mix of wild-type (CD45.1 + ) and CD27 −/− (CD45.2 + ) T-cell-depleted bone-marrow cells. Eight weeks after reconstitution, the chimeras were primed with 5×10 6 Act-mOVA/K b−/− splenocytes and challenged at day 40 with 5×10 6 pfu Vacc-OVA. The frequency of OVA 257−264 /K b –specific CTL of each type at primary, memory and following secondary expansion in the presence (helped) versus absence (helpless) of CD4 + T cells is shown. Standard error bars represent the s.d. of mice in each group. Significant difference was calculated by an unpaired two-tailed t -test. * P -value<0.05; ** P <0.005; *** P <0.0005. Figure shows representative experiments that were repeated at least twice with similar results. Full size image CD27 −/− CTL have reduced numbers of memory precursors We next investigated the functional and phenotypic consequences of CD27 signalling on CTL function. CD27 is not strictly required for development of effector function as both endogenous and transgenic CTL lacking CD27 were able to eradicate target cells in vivo ( Fig. 5a,b ). The absence of CD27 on CTL did, however, lead to a pronounced decrease in their ability to produce IL-2 on antigenic reencounter at the memory stage ( Fig. 5c ). This confirms data from previous studies [24] , [27] demonstrating that CD27 signalling enhances autocrine IL-2 production. A decrease in the frequency of cells producing IFN-γ on exposure to antigen in vitro during the secondary response was observed in CD27-deficient CD8 + T cells ( Fig. 5d ). Lastly, we noted a reduction in the frequency of CD8 + T cells expressing the memory precursor effector cell phenotype among those lacking CD27 ( Fig. 5e ), although the relative frequency of CTL expressing the effector memory (CD127 + CD62L − ) versus central memory surface phenotype did not differ between wild-type and CD27-deficient CD8 + T cells, despite the secondary expansion defect displayed when they lacked CD27 ( Fig. 5f ). Taken together, these data reveal that CTL lacking CD27 display distinct alterations in their functional capacity, most notably a failure to generate multifunctional effectors capable of autocrine IL-2 production in the memory response. 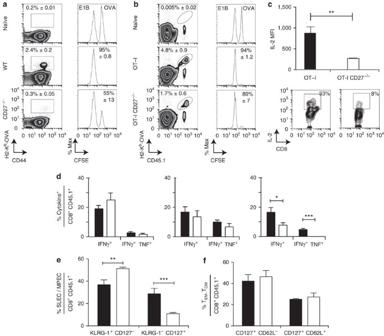Figure 5: CD27 influences functional and phenotypic characteristics. (a,b)In vivocytotoxicity assays were performed in (CD45.2+) WT or CD27−/−mice in (a), or in WT mice injected with 5,000 WT or CD27−/−OT-I (CD45.1+) cells in (b), 5 days after Act-mOVA/Kb−/−challenge. (c,d) Groups of 4–5 C57BL/6 mice received 50 WT or CD27−/−OT-I CD8+ T cells (CD45.1+) were injected in WT mice. One day later, the mice were challenged with 5×106Act-mOVA/Kb−/−splenocytes. The primary response was measured after 7 days. The mice were rechallenged 30 to 40 days later with 5×106pfu Vacc-OVA and the response was measured 5 days later. (c) Autocrine IL-2 production was measured by intracellular cytokine staining in memory WT and CD27−/−OT-I cells restimulated with OVA257−264peptide, 40 days after priming. Mean Fluorescence Intensity (MFI) for both populations is shown. (d) The frequency of IFNγ+and IFNγ+TNF+cells among the total OT-I (black bars) or OT-I CD27−/−(white bars) population during the primary, memory and secondary response is shown. The cytokines were measured by intracellular staining after 5 h restimulation with OVA257−264peptide in presence of brefeldin A. (e) The frequency of OT-I (black bars) or OT-I CD27−/−(white bars) cells bearing the SLEC (KLRG1+CD127−) and memory precursor effect cell (KLRG1−CD127+) surface phenotype 5 days after priming. (f) The frequency of OT-I (black bars) or OT-I CD27−/−(white bars) cells expressing the effector memory (CD127+CD62L−) and central memory (CD127+CD62L+) surface phenotype 40 days after priming. Error bars represent s.d. of 3–4 mice. Significance was calculated by a two-tailed unpairedt-test. *P-value<0.05; **P<0.005; ***P<0.0005. Figure shows representative experiments that were repeated at least twice with similar results. Figure 5: CD27 influences functional and phenotypic characteristics. ( a , b ) In vivo cytotoxicity assays were performed in (CD45.2 + ) WT or CD27 −/− mice in ( a ), or in WT mice injected with 5,000 WT or CD27 −/− OT-I (CD45.1 + ) cells in ( b ), 5 days after Act-mOVA/Kb −/− challenge. ( c,d ) Groups of 4–5 C57BL/6 mice received 50 WT or CD27 −/− OT-I CD8+ T cells (CD45.1 + ) were injected in WT mice. One day later, the mice were challenged with 5×10 6 Act-mOVA/K b−/− splenocytes. The primary response was measured after 7 days. The mice were rechallenged 30 to 40 days later with 5×10 6 pfu Vacc-OVA and the response was measured 5 days later. ( c ) Autocrine IL-2 production was measured by intracellular cytokine staining in memory WT and CD27 −/− OT-I cells restimulated with OVA 257−264 peptide, 40 days after priming. Mean Fluorescence Intensity (MFI) for both populations is shown. ( d ) The frequency of IFNγ + and IFNγ + TNF + cells among the total OT-I (black bars) or OT-I CD27 −/− (white bars) population during the primary, memory and secondary response is shown. The cytokines were measured by intracellular staining after 5 h restimulation with OVA 257−264 peptide in presence of brefeldin A. ( e ) The frequency of OT-I (black bars) or OT-I CD27 −/− (white bars) cells bearing the SLEC (KLRG1 + CD127 − ) and memory precursor effect cell (KLRG1 − CD127 + ) surface phenotype 5 days after priming. ( f ) The frequency of OT-I (black bars) or OT-I CD27 −/− (white bars) cells expressing the effector memory (CD127 + CD62L − ) and central memory (CD127 + CD62L + ) surface phenotype 40 days after priming. Error bars represent s.d. of 3–4 mice. Significance was calculated by a two-tailed unpaired t -test. * P -value<0.05; ** P <0.005; *** P <0.0005. Figure shows representative experiments that were repeated at least twice with similar results. Full size image CD27 transmits the 'help message' to CTL The cumulative results described above suggest that interfering with CD27–CD70 interactions prevents transmission of the help message to CTL, leading to a functionally equivalent state of 'helplessness' to that which occurs when they are primed in the absence of T H cells. A central feature of this condition is the induction of TRAIL-mediated AICD on secondary stimulation of helpless CD8 + T cells. To determine whether TRAIL similarly controls the secondary expansion defect induced in the absence of CD27 signals to CTL, we generated OT-I mice lacking expression of both CD27 and TRAIL and performed adoptive transfer experiments using intact or CD4-depleted C57BL/6 mice as recipients that were subsequently immunized with Act-mOVA/K b−/− splenocytes. As expected, in vitro secondary expansion of OT-I depended on the presence of CD4 + T cells during in vivo priming but was restored when the OT-I cells lacked the TRAIL gene ( Fig. 6a,b ). Consistent with the cumulative data on in vivo secondary responses, the absence of CD27 on the OT-I cells prevented them from receiving the necessary signals to enable their secondary expansion ( Fig. 6c,d ). When the TRAIL gene was also absent from the CD27 −/− OT-I; however, their defective secondary response was restored. These data demonstrate that CTL deprived of CD27 signals are functionally and phenotypically equivalent to the helpless cells generated in the absence of CD4 + T cells and suggest the existence of a molecular link between CD27 signals and the downstream regulation of secondary expansion by TRAIL expression. Taken together, our studies show that CD27 is the receptor through which the 'T cell help' signal is transmitted to CTL during priming. 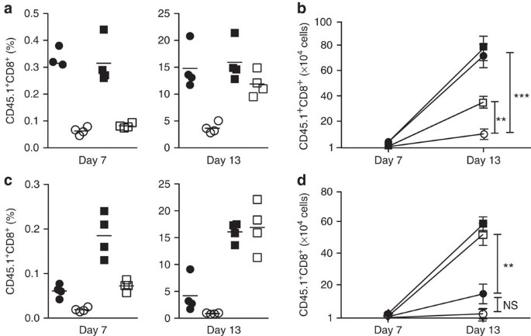Figure 6: TRAIL controls the helpless phenotype in absence of CD27. (a,b) Groups of wild-type C57BL/6 mice (filled symbols) or CD4-depleted mice (open symbols) received 50 OT-I WT CD45.1+(circles) and 50 OT-I TRAIL−/−CD45.1+/2+(squares) and were challenged 1 day later with 5×106Act-mOVAKb−/−splenocytes. The primary response was measured 7 days later by CD45.1+/2+staining before re-stimulation with MEC.B7.SigOVA cells. Secondary expansion of OVA-specific CTL was measured by the same method 6 days later. (a) The percentage of OT-I CD8+ among total splenocytes with the average value depicted by the horizontal line, and (b) their absolute number. (c,d) Groups of wild-type C57BL/6 mice (filled symbols) or CD4-depleted mice (open symbols) 50 OT-I CD27−/−CD45.1+(circles) and 50 OT-I CD27−/−TRAIL−/−CD45.1/2+(squares) and were challenged and re-stimulated, as described above. Significant difference was calculated by an unpaired two-tailedt-test. *P-value <0.05; **P<0.005; ***P<0.0005. Figure shows representative experiments that were repeated at least twice with similar results. NS, not significant. Figure 6: TRAIL controls the helpless phenotype in absence of CD27. ( a , b ) Groups of wild-type C57BL/6 mice (filled symbols) or CD4-depleted mice (open symbols) received 50 OT-I WT CD45.1 + (circles) and 50 OT-I TRAIL −/− CD45.1 + /2 + (squares) and were challenged 1 day later with 5×10 6 Act-mOVAK b−/− splenocytes. The primary response was measured 7 days later by CD45.1 + /2 + staining before re-stimulation with MEC.B7.SigOVA cells. Secondary expansion of OVA-specific CTL was measured by the same method 6 days later. ( a ) The percentage of OT-I CD8+ among total splenocytes with the average value depicted by the horizontal line, and ( b ) their absolute number. ( c , d ) Groups of wild-type C57BL/6 mice (filled symbols) or CD4-depleted mice (open symbols) 50 OT-I CD27 −/− CD45.1 + (circles) and 50 OT-I CD27 −/− TRAIL −/− CD45.1/2 + (squares) and were challenged and re-stimulated, as described above. Significant difference was calculated by an unpaired two-tailed t -test. * P -value <0.05; ** P <0.005; *** P <0.0005. Figure shows representative experiments that were repeated at least twice with similar results. NS, not significant. Full size image This study provides the first evidence for the cognate interaction between APC and CTL cells that endow the latter with the capacity for secondary expansion and avoidance of TRAIL-mediated AICD, both of which are essential functional components of the memory state [6] , [7] , [8] , [9] . Although previous studies have indicated a role for soluble factors such as CCL3/CCL4, IL-15 and IL-21 as underlying the requirement for CD4 + T cells in the generation of optimal CTL responses, none have defined a specific alteration in the stimulatory capacity of APC activated via CD40 engagement by CD4 + T cells that enables transmission of a distinct signal to CTL through which they can acquire the capacity for proliferative recall responses [28] , [29] , [30] , [31] , [32] . Our studies break new ground in this regard with the demonstration that, following vaccination with either a noninflammatory nonreplicating antigen (cross-primed cellular vaccines) or an overtly inflammatory replicating antigen (vaccinia virus and Listeria monocytogenes) , CTL, prevented from receiving a signal through CD27 during priming, subsequently exhibit a specific defect in their capacity for secondary expansion ( Figs 1 , 2 , 3 , 4 ). This outcome is seen with both the endogenous polyclonal repertoire as well as with monoclonal transgenic CTL in single- and double-transfer settings in which the endogenous (wild-type) response can be monitored side by side with the transferred population. Additionally, we observe the same outcome in bone-marrow chimeras in which wild-type and CD27-deficient CTL can similarly be measured simultaneously ( Fig. 4 ). Thus, with a range of immunogens, responding T cells, and blocking strategies, the absence of CD27 signals to CD8 + T cells prevents their developing the capacity for secondary proliferative responses. Our finding that this defect is relieved in the absence of TRAIL expression shows a common link between helpless CD8 + T cells and those denied CD27 signals during priming in the presence of T cell help. As both the primary and secondary responses of CD8 + T cells primed in the absence of both CD4 + T cells and CD27 signals was lower than CD27 + wild-type cells similarly primed under 'helpless' conditions alone, our data suggest that CD27–CD70 signals alone are unlikely to constitute the entire contribution of CD4 + T cells to the priming and maintenance of CD8 + T cells, consistent with previous reports 1,5 . As the levels of CD70 on CD11c + APC from CD4-depleted mice are only slightly lower than in wild-type mice, our data further suggest that CD4 + T cells are unlikely to be the only factor capable of maintaining its expression on DC. Nonetheless, preventing the interaction of CD70 with CD27 on CD8 + T cells resulted in a cell-intrinsic defect in secondary proliferation, underscoring the importance of this pathway in transmitting the help message from activated APC to CTL. Previous studies have suggested that the requirement for CD27 expression on CD8 + T cells, to enable their optimal primary and secondary responses, depends on the immunogen used, but none has so far related this pathway to the provision of T H cells and the prevention of TRAIL-mediated AICD [6] , [17] , [18] , [21] , [33] , [34] . Our combined results demonstrate for the first time that, in circumstances where CD4 + T cell help can be shown to be both essential for secondary expansion and is amply provided, the absence of CD27 alone on CTL prevents them from acquiring the 'helped' state. This is further confirmed by our finding that relieving both helpless and CD27-deficient CTL from TRAIL-mediated AICD restores their ability to undergo secondary expansion ( Fig. 6 ). This observation provides confirmation that CD27 signals constitute the 'help' signal received by CTL, and suggests that a critical downstream consequence of this is to engage the mechanism that prevents transcriptional activation of TRAIL on restimulation of helpless CTL. This insight offers a useful starting point for identifying the intracellular signalling pathways linking membrane engagement of CD27 with downstream signal transduction and gene-regulation events that control the selective induction of TRAIL expression in helpless cells. It is notable that CD8 + T cells lacking CD27 produce substantially less IL-2 than their wild-type counterparts [24] , [27] , and we have previously shown that IL-2 can overcome the secondary expansion defect displayed by helpless cells [6] , [35] , [36] . In summary, our findings identify the CD27/CD70 pathway as that which allows APC activated by CD4 + T cells to program CD8 + T cells with the capacity for secondary expansion, and complete our understanding of the cellular interactions through which T - cell help establishes a memory state in CD8 + T cells [28] , [29] , [31] , [32] . As CD8 + T cells have a key role in a range of immune responses, these insights should lead to new opportunities for therapeutic intervention in cancer, autoimmunity, transplantation and infectious disease, with elucidation of the molecular pathways that link CD27 engagement to the gene expression events that regulate secondary expansion providing additional targets for this goal. Mice C57BL/6J mice were purchased from The Jackson Laboratory. CD27 −/− , OT-I Rag −/− CD45.1 + and Act-mOVA/Kb −/− mice on a C57BL/6J background have been previously described [21] , [37] . OT-I Rag −/− CD27 −/− CD45.1 + mice were generated by intercrossing CD27 −/− with OT-I Rag −/− CD45.1 + . The OT-II CD27 −/− mice were generated by intercross with CD27 −/− with OT-II. Mice were maintained by in-house breeding at the La Jolla Institute for Allergy and Immunology under specific pathogen-free conditions, in accordance with guidelines by the Association for Assessment and Accreditation of Laboratory Animal Care International. Immunizations At the time points and frequency described in the figure legends and text, groups of mice were either primed with 5×10 6 Act-mOVA/Kb −/− splenocytes intravenously and were challenged intraperitoneally with 5×10 6 pfu Vacc-OVA (VACV-WR-OVA strain) or were primed with 1×10 6 pfu Vacc-OVA and challenged intravenously with 0.6. LD50 Listeria-OVA. Antibody treatment Depletion of CD4 + cells in vivo was performed by intraperitoneal administration of 200 and 100 μg of GK1.5. antibody, respectively, 3 and 1 day before immunization for the 'helpless' groups; 4 days after immunization, 200 or 100 μg GK1.5 was administrated, respectively, to the 'helped' and 'helpless' groups. The blocking of CD70 (FR70) was performed by intraperitoneal administration of 250 μg at day −1, 0 and 3 of immunization. The control mice were injected with a Rat IgG isotype control (Chemicon International). T-cell preparations For transfer of OT-I CD45.1 + cells or OT-I CD27 −/− , CD45.1 + , OT-I Rag −/− CD45.1 + mice were bled, and the number of OT-I cells was determined by counting and by fluorescence-activated cell sorting (FACS) staining for Vα2 + Vβ5 + . 50 OT-I cells were injected per mouse, given intravenously admixed with 1–2×10 6 LCMV P14 CD90.1 + splenocytes used as an internal reference control for the transferred cell population for FACS acquisition. For co-transfer of OT-I CD27 −/− CD45.1 + and OT-I CD45.1/2 + , OT-I Rag −/− mice were bled, and the number of OT-I cells was determined by counting and FACS staining for Vα2 + Vβ5 + . 50 OT-I CD27 −/− CD45.1 + plus 50 OT-I CD45.1/2 + cells per mouse were injected intravenously. For transfer of OT-II cells, CD4 + splenocytes were negatively selected (MACS, Miltenyi). The number of OT-II cells was determined by counting and by FACS staining for Vα2 + Vβ5 + . 50,000 OT-II cells were injected intravenously. Ex-vivo re-stimulation and antibody staining Cytokine production in CD8 + T cells was assessed as described: splenocytes from immunized mice were resuspended in IMDM medium (Invitrogen) supplemented with 8% FCS (Omega Scientific), 1% L -glutamine (Invitrogen), 100 μg ml −1 streptomycin, 100 U ml −1 penicillin, and 50 μM 2-ME (Sigma-Aldrich). Cells (1–2×10 6 ) were plated in 96-well round-bottom plates in case of Act-mOVA/Kb −/− and Vacc-OVA stimulation or in 96-well flat bottom plates in the case of listeria-OVA in 200 μl medium plus OVA peptide 357–364 (SIINFEKL peptide) at 1 μg ml −1 in presence of GolgiPlug (BD Biosciences) for 5 h at 37 °C. Cells were stained with anti-CD8 (PE-TR, 0.05 μg per 10 6 cells), CD62L (Alexa-Fluor 750, 0.05 μg per 10 6 cells), CD27 (FITC, 0.1 μg per 10 6 cells), CD44 (Alexa-Fluor 700, 0.05 μg per 10 6 cells), CD45.1 (Pacific Blue, 0.05 μg per 10 6 cells) and CD45.2 (Percp-Cy5.5, 0.1 μg per 10 6 cells) followed by fixation with Cytofix-Cytoperm (BD Biosciences) for 20 min at 4 °C. Fixed cells were subjected to intracellular cytokine staining in Perm/Wash buffer (BD Biosciences) for 30 min at 4 °C. Anti-TNF (Pe-cy7, 0.1 μg per 10 6 cells), IFNγ (APC, 0.05 μg per 10 6 cells) and IL-2 (PE, 0.1 μg per 10 6 cells). The antibodies were purchased from BD Pharmingen, eBiosciences or BioLegend. The samples were acquired on a LSRII flow cytometer (Becton Dickinson) and analysed using FlowJo software. Tetramer staining and flow cytometry Cells were stained with directly conjugated OVA/Kb tetramer (PE) (BD Pharmingen) at room temperature for 10 min followed by antibody staining with anti-CD8 (PE-TR, 0.05 μg per 10 6 cells), CD62L (Alexa-Fluor 750, 0.05 μg per 10 6 cells), CD27 (FITC, 0.1 μg per 10 6 cells), CD44 (Alexa-Fluor 700, 0.05 μg per 10 6 cells), CD127 (APC, 0.05 μg per 10 6 cells) and KLRG-1 (Pe-Cy7, 0.05 μg per 10 6 cells). The antibodies were purchased from BD Pharmingen, eBiosciences or BioLegend. The samples were acquired on an LSRII flow cytometer (Becton Dickinson) and analysed using FlowJo software. In vivo cytotoxic assay The cytotoxic assay was performed in the endogenous system or in the transgenic system. In both cases, the mice were immunized, at day 0, with 5×10 6 Act-mOVA/Kb −/− splenocytes intravenously. At day 5, 5×10 6 of CD45.1 + splenocytes loaded with Ski9 peptide (irrelevant peptide) and 5×10 6 of CD45.1 + splenocytes loaded with OVA peptide 357–364 (relevant peptide) stained, respectively, with 0.02 and 0.2 μM CFSE were injected intravenously. 15 h later, the spleens were removed. The samples were acquired on a LSRII flow cytometer (Becton Dickinson) and analysed using FlowJo software. Dendritic cell preparation and flow cytometry Spleens from immunized or naïve mice were perfused with 1 mg ml −1 collagenase D in presence of DNAse I. After perfusion, the spleens were cut in small pieces and incubated for 30 min at 37 °C. The cells were then put in suspension and washed. The samples were then blocked with 24G2 to block the Fc receptors for 10 min at 4 °C, followed by antibody staining with anti-CD11c (PECy7, 0.1 μg per 10 6 cells), CD11b (APC, 0.1 μg per 10 6 cells) and CD70 (PE, 0.1 μg per 10 6 cells). The antibodies were purchased from BD Pharmingen or eBiosciences. The samples were acquired on an LSRII flow cytometer (Becton Dickinson) and analysed using FlowJo software. How to cite this article: Feau, S. et al . The CD4 + T-cell help signal is transmitted from APC to CD8 + T-cells via CD27–CD70 interactions. Nat. Commun. 3:948 doi: 10.1038/ncomms1948 (2012).